Ordered macroporous platinum electrode and enhanced mass transfer in fuel cells using inverse opal structure Three-dimensional, ordered macroporous materials such as inverse opal structures are attractive materials for various applications in electrochemical devices because of the benefits derived from their periodic structures: relatively large surface areas, large voidage, low tortuosity and interconnected macropores. However, a direct application of an inverse opal structure in membrane electrode assemblies has been considered impractical because of the limitations in fabrication routes including an unsuitable substrate. Here we report the demonstration of a single cell that maintains an inverse opal structure entirely within a membrane electrode assembly. Compared with the conventional catalyst slurry, an ink-based assembly, this modified assembly has a robust and integrated configuration of catalyst layers; therefore, the loss of catalyst particles can be minimized. Furthermore, the inverse-opal-structure electrode maintains an effective porosity, an enhanced performance, as well as an improved mass transfer and more effective water management, owing to its morphological advantages. Hydrogen is the most abundant element on Earth. It can be converted into non-polluting, zero-emission renewable energy, it is unlikely to be subject to geopolitical pressures or scarcity concerns, and it does not contribute to global warming through CO 2 emissions. It shows good performance in fuel cells, which can have 2.5 times the efficiency of internal combustion engines [1] . Consequently, such fuel cells are considered a promising future technology for energy conversion [2] , [3] . Among the various kinds of fuel cells, polymer electrolyte membrane fuel cells (PEMFCs) are the most encouraging for commercial applications. However, the key factor in fuel cell performance is the structure of the electrode in the membrane electrode assembly (MEA). Hence, optimization and modification of electrode structure have proven to be critical for improving the performance and durability of PEMFCs [4] , [5] . Accordingly, several attempts have been made to enhance mass transfer and improve water management through careful design of the electrode structure, for example, the use of an additional solvent to control the polarity [6] , [7] , [8] , application of a pore-forming agent [9] , and optimization of the ionomer content [10] . Furthermore, three-dimensional (3D) nanostructured materials have been introduced for catalyst supports including carbon nanotubes, carbon nanofibers, layer-by-layer assemblies and inverse opal structures [11] , [12] , [13] , [14] , [15] . However, ordered, carbon-based catalyst supports such as carbon nanotubes are acquired through a difficult, costly fabrication process. Moreover, the corrosion and oxidation of carbon supports is also a major problem that can restrict the durability of the catalyst [16] , [17] , [18] , [19] . The loss of catalytic Pt particles within a catalyst layer can occur in conventional catalyst slurry (ink-based MEA). This has prompted the formation of catalyst layers that consist of carbon-supported Pt particle clusters and ionomer aggregations by a random bottom-up approach. Accordingly, balancing these conflicting and inter-related requirements remains an intricate problem, and the fabrication of a satisfactory, ordered nanostructured electrode has not yet been achieved. Therefore, finding ways to improve upon these current methods is a major priority. Mass transport in a fuel cell is affected by convection in flow channels and diffusion across electrodes. Electrochemical reactions on one side of an electrode, and convective mixing on the other side of the electrode, cause concentration gradients leading to diffusive transport across the electrode. Diffusional flux and limiting current are affected by the effective diffusivity, electrode thickness and tortuosity [20] . Moreover, not all of the catalysts used to construct the fuel cell electrodes are accessible to reactants (for example, protons and oxygen). In disorderly structured electrodes such as conventional MEAs ( Fig. 1a ), gas molecules tend to be impeded by pore walls and other particles; therefore, the effective diffusivity is lower than that for an inverse-opal-structure Pt electrode (denoted hereafter as an IO electrode, Fig. 1b ). However, an IO electrode shows enhanced mass diffusivity resulting from its open and interconnected pore architecture, and it is possible to produce a thinner electrode. In addition, this electrode is free from the release of disconnected particles, owing to robust and wholly integrated catalyst layer structures. 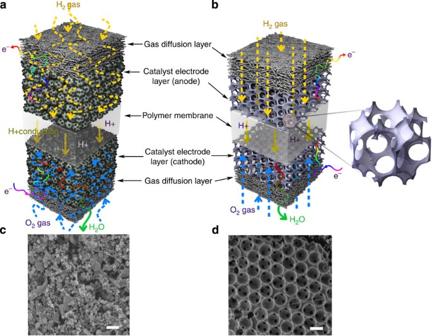Figure 1: Conceptual diagrams of two MEAs. (a) Conventional MEA with CCM, (b) modified MEA with inverse-opal-structure (IO) electrode examined in this study. (c) FE-SEM image of a CCM surface prepared by commercial Pt/C ink spraying. (d) FE-SEM image of an IO electrode surface prepared by pulse electrodeposition according to colloidal crystal templating methods. Scale bar, 500 nm. Figure 1: Conceptual diagrams of two MEAs. ( a ) Conventional MEA with CCM, ( b ) modified MEA with inverse-opal-structure (IO) electrode examined in this study. ( c ) FE-SEM image of a CCM surface prepared by commercial Pt/C ink spraying. ( d ) FE-SEM image of an IO electrode surface prepared by pulse electrodeposition according to colloidal crystal templating methods. Scale bar, 500 nm. Full size image Template fabrication using self-assembled closely packed colloidal spheres is a general method of preparing 3D-ordered macroporous (3DOM) materials [21] , [22] , [23] , [24] , [25] . Such ordered materials have previously been investigated for potential use in various applications, including photonic crystals, optical sensors, catalysts, capacitors, dye-sensitized solar cells, battery materials and fuel cells [26] , [27] , [28] , [29] , [30] , [31] , [32] . This is because of the benefits that result from the periodic structure of ordered materials, their relatively large surface areas and their interconnected macropores. For example, if a 3DOM material is introduced into an electrochemical device, such as an MEA in a PEMFC ( Fig. 1b ), the morphological advantages from the open surface and interconnected pore architecture of electrodes are manifold. Firstly, the architecture consists of highly open, short diffusion pathways with reduced resistance and low tortuosity, which facilitate improved mass transport and increased conductivity compared with a tortuous structure. Secondly, the architecture also has a larger interfacial area, on which the electrode reaction can occur, and an increased number of active sites per unit MEA area, which leads to an improvement in the apparent reaction rate. Thirdly, the architecture also exhibits reduced thickness leading to increased conductivity of both reactants and ions, so that the ionomer can be unnecessary. Finally, the architecture also exhibits interconnected grains that result in a reduced release of disconnected particles into the surrounding environment. Thus, it has been demonstrated that 3DOM materials can enhance the performance of an individual electrode [33] . Nevertheless, the application of inverse opal materials to electrodes in fuel cells has been limited to solid oxide fuel cells [34] , [35] , [36] , and applications in PEMFCs have been restricted to only a small number of components. This is probably the result of the significant limitations in fabrication routes for inverse opal materials. Most notably, the ideal substrate for self-assembly of colloidal spheres is a planar, non-porous and chemically homogeneous surface; yet, most active devices such as gas diffusion layers (GDLs) and polymer membranes in PEMFCs with rough surfaces, are chemically heterogeneous and often porous [37] . Because of these properties, the direct application of an IO electrode in MEAs in PEMFCs has been considered impractical. Without an additional transfer process, a single cell that maintained an inverse opal structure entirely within an MEA was considered impossible. Previous attempts to introduce an inverse opal structure into PEMFCs have been limited to the electro catalysis of half-cells [38] , [39] , [40] , [41] , catalyst supports [11] , [12] , [13] , [14] , [15] , [16] , [17] , [18] , [19] , or membranes [42] , [43] , [44] . To the best of our knowledge, there have been no reports on their practical use as electrodes, or on their single-cell performance; thus, the benefits arising from their structure have not been properly determined. Here we report a direct application of an IO electrode to MEAs in PEMFCs, without any additional transfer process at the electrodes. This is achieved using electrodeposition following colloidal crystal templating methods. Furthermore, the performance of an IO electrode is demonstrated in a practical device. The enhanced mass transfer of an IO electrode and its characteristic performance are also discussed. Self-assembly of polystyrene beads A schematic diagram illustrating the fabrication of an IO electrode and the corresponding field-emission scanning electron microscopy (FE-SEM) images of the latter are shown in Fig. 2 . Most substrates that have been used for template fabrication of IO structures have had flat and even surfaces, for example, glass slides, Si wafers, indium tin oxide and fluorine-doped tin oxide. However, in the present study, GDLs containing microporous layers (MPLs; 35BC and SGL), which are generally used as GDLs in PEMFCs, were used as substrates to directly apply an IO structure into MEAs, without an additional electrode transfer process. The MPLs consist of carbon black and 5 wt% of polytetrafluoroethylene; thus, the surfaces of MPLs are rough and uneven compared with those of the substrates used in previous studies. Consequently, a simple substrate pretreatment must be performed before polystyrene (PS) bead deposition. Atomic force microscopy images and corresponding FE-SEM images for the surface morphology of pristine GDL are shown in Supplementary Fig. S1 . The surface is jagged and rough because of carbon black particles agglomerating together to form larger clusters. However, the number of void spaces on the GDL surface is negligible compared with the size of colloids used for templating. The GDLs were soaked in a solution of 1,2-ethanedithiol in ethanol to enhance adhesion between the substrate and the colloid. It was not possible to deposit PS beads onto the GDLs without the presence of MPLs (for example, GDLs of Toray, Japan), as there was a lack of carbon and alkanethiols on the substrate surface, although they were prepared using the same pretreatment. The formation of self-assembled monolayers of thiols on gold surfaces is well known, but there have only been a few studies reported on the adsorption of organic thiols on carbon. However, carbon black has a surface with energetic heterogeneity, and the most active sites are graphite edges [45] , [46] . As a consequence, alkanethiols will be adsorbed spontaneously along the edges of a crystal by oxidative addition and reductive elimination of head-thiol groups. These adsorbed alkanethiols can act as a type of binder or coupling agent by interacting with the carboxyl groups on the PS surface and the terminal-thiol groups on the carbon black surface. In the present study, 0.5 wt% of non-ionic surfactant was added to a PS colloid suspension to facilitate self-assembly and crystallization of the PS beads. When added in water, surfactant molecules strongly positively adsorb at the PS bead surfaces, changing the properties of the suspension, including its hydrophilicity and surface tension. PS particles were self-assembled, and a structured crystal template was produced by water evaporation and sequential convective flux during vertical deposition [47] , [48] , [49] . When the water was evaporated from the meniscus, particles were continuously transported to the vicinity of the triple-phase contact line by convective fluid flow of the surrounding suspension. Simultaneously, capillary forces in the drying film pulled the spheres together to form an ordered, closely packed structure ( Fig. 2b ). A more uniform surface with fewer defects was obtained by diluting the PS suspension with ethanol, whereas faster evaporation resulted in a thicker template. The thickness of the template was controlled by modifying the solvent evaporation rate or the solution concentration; a related equation with other parameters has previously been reported to explain this phenomenon [49] . 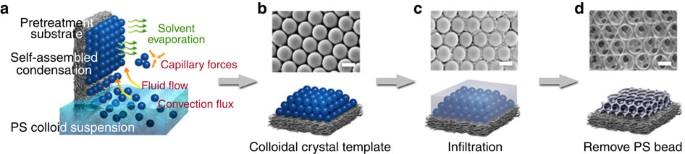Figure 2: Schematic diagram of the fabrication process. (a) Vertical deposition of PS beads on a pretreated substrate (GDL). (b) Self-assembly of a colloidal crystal template on GDL. (c) Infiltration and pulse electrodeposition. (d) Removal of colloidal crystal template by soaking in toluene. Scale bar, 500 nm. Figure 2: Schematic diagram of the fabrication process. ( a ) Vertical deposition of PS beads on a pretreated substrate (GDL). ( b ) Self-assembly of a colloidal crystal template on GDL. ( c ) Infiltration and pulse electrodeposition. ( d ) Removal of colloidal crystal template by soaking in toluene. Scale bar, 500 nm. Full size image Fabrication of IO Pt electrode and MEA For Pt infiltration into a PS template, galvanostatic-pulsed electrodeposition onto the template was performed. The corresponding results and SEM images of the GDL surface are shown in Fig. 2c . Also, large-area SEM images of the IO electrode are shown in Fig. 3 . The GDL substrate under the template served as a working electrode. Pulsed electrodeposition was used because this method has the distinct advantage of improving the physical properties of the deposit and its adherence to the substrate. In addition, nucleation and growth can be controlled separately by adjusting the potential pulse amplitudes and the duration of deposition [50] . The current density, duty cycle and charge density were changed to produce an electrode surface with better morphology ( Supplementary Fig. S2 and Supplementary Note 1 ). The total charge density was fixed at 4 C cm −2 , which implies that the theoretical Pt loading was 0.2 mg cm −2 . However, the actual amount of Pt deposited onto the GDL was ~0.12 mg cm −2 , as determined using inductively coupled plasma (ICP) mass spectrometry. The thickness of each IO electrode was ~1–2 μm ( Fig. 4 ); therefore, a total charge of 1 C cm −2 was deposited, corresponding to a Pt deposit of 0.03 mg cm −2 and a thickness of ~0.5 μm. PS spheres were deposited with 5–20 layers on GDL and the corresponding thickness was ~3–12 μm. In the case of the inverse-opal-structure Pt spheres, the thickness was ~3–4 layers (1.5–2 μm). The thickness was determined by considering the restricted Pt amounts, the preserved IO structure and the smooth proton transfer. Considering that typical thickness values of conventional electrodes in PEMFCs are ~5–10 μm, the IO electrode is superior to conventional electrodes having a shorter diffusion path and increased conductivity of the reactants and ions, which means that the use of an ionomer for proton transfer is unnecessary. 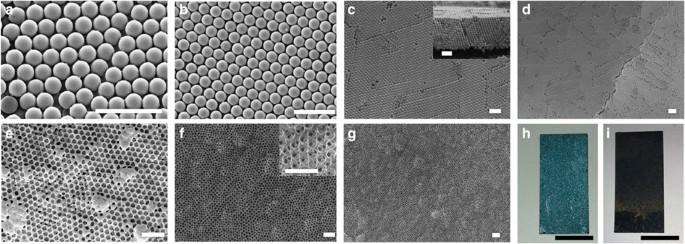Figure 3: FE-SEM images of electrodes. (a–d) PS crystal template on GDLs (inset ofc: cross-sectional image); scale bars, 2 μm. (e–g) IO electrodes on GDLs (inset off: closer look); scale bars, 2 μm. (h,i) Photograph of actual electrode on GDL after PS deposition (h) and PS removal (i) following electrodeposition; scale bars, 2 cm. Figure 3: FE-SEM images of electrodes. ( a – d ) PS crystal template on GDLs (inset of c : cross-sectional image); scale bars, 2 μm. ( e – g ) IO electrodes on GDLs (inset of f : closer look); scale bars, 2 μm. ( h , i ) Photograph of actual electrode on GDL after PS deposition ( h ) and PS removal ( i ) following electrodeposition; scale bars, 2 cm. 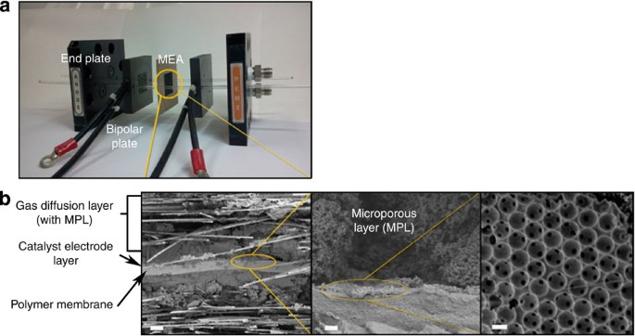Figure 4: Photograph of practical PEMFC single cell. (a) MEA in single cell is used for this study. (b) Cross-sectional FE-SEM images of MEA with inverse-opal-structure (IO) electrode on GDL (scale bars, 50 μm, 2 μm and 500 nm, respectively). Full size image Figure 4: Photograph of practical PEMFC single cell. ( a ) MEA in single cell is used for this study. ( b ) Cross-sectional FE-SEM images of MEA with inverse-opal-structure (IO) electrode on GDL (scale bars, 50 μm, 2 μm and 500 nm, respectively). Full size image An inverse duplicate of the hexagonal close-packed structure, which has a packing factor of 0.74, consists of closely packed planes of PS beads. For the opal-structure template, the skeletal walls enclose macropores that are interconnected through holes at the points where the original PS beads touch. Indeed, the structure of inversed opal materials, which are obtained from electrodeposition based on colloidal crystal templating methods, is usually formed by filling the interstitial spaces of the template with the desired materials. However, this phenomenon was not observed in this study. Instead, Pt surrounds the PS spheres creating a shell ( Figs 1b and 2d ). The thickness of the Pt walls was determined to be ~10–15 nm, and this was calculated using SEM images and approximate calculations of the surface ratio (see Supplementary Note 1 for details). X-ray diffraction analysis was performed to verify the presence of the Pt component on the IO electrode ( Supplementary Fig. S3 ). Three major peaks at 40.06, 46.54 and 67.86° in the spectrum correspond to Pt(111), (200) and (220) planes, respectively. Characteristic peaks at ~27° arise from the carbon in the MPL of the GDL. The size of the Pt grains that formed on the IO electrode-based MEA was calculated to be ~8–11 nm using the Scherrer equation and X-ray diffraction data. In addition, to further characterize the surface Pt of the IO electrode, X-ray photoelectron spectra (XPS) ( Supplementary Fig. S4 ) were obtained. The oxidation states of Pt in the IO electrode are quite different from those in conventional Pt/C electrodes. The XPS spectra in Supplementary Fig. S4 show that the Pt 4f core-level peaks of Pt/C of the conventional electrode are mainly derived from Pt(0), but in the case of the IO Pt electrode, the main peak comes from Pt(II). In addition, the distribution of Pt oxidation states in the IO electrode is different from that of Pt/C in the conventional electrode ( Supplementary Fig. S5 and Supplementary Table S1 ). However, these observations are not of major relevance to the performance of the cell, as the oxidation state of the Pt surface is susceptible to heat treatment conditions and easily changes during the cell operation [4] . A modified MEA was fabricated using the electrodeposited IO electrode as a cathode to test the performance of the IO electrode in a practical device ( Fig. 4 ). The ionomer in the catalyst layer serves as a binder, proton conductor and hydrophilic agent, and it improved the catalyst utilization [51] . Nevertheless, the ionomer was unnecessary for the IO electrode in this study. In addition, although there were no ionomers in the cathode catalyst, the performance did not decrease because of the geometrical advantages of the IO structure and the short diffusion pathway of the thinner electrode. Moreover, the active area of the electrode was 5 cm 2 , which was a relatively large area in the case of IO structure applied materials [23] . In the fuel cell system, the dead-end mode requires neither fuel nor an oxidant supplying device, such as a blower, fan or recirculation unit; therefore, improved efficiency and a simplified system are expected [52] . Thus, in addition to standard fuel cell test condition from US Department of Energy’s reference, the cathodic dead-end mode was also used with the IO electrode to widen its potential use in applications such as micro fuel cells. Performance of IO electrode-based MEA The polarization and power density curves for two MEAs are shown in Fig. 5 . They were measured in cathode dead-end mode with a fully humidified gas at 70 °C ( Fig. 5a ) and under ambient humidity at room temperature ( Fig. 5b ). 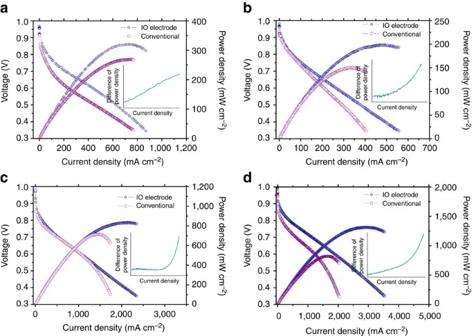Figure 5: Polarization curves of IO electrode-based MEAs. (a) Using a fully humidified H2/O2supplement and maintained at 80 °C. (b) Under ambient humidity and room temperature condition. For both MEAs, the cathode catalyst loading was ~0.12 mg cm−2. (c) Polarization curves from US Department of Energy’s reference conditions with 0.12 mg cm−2and (d) 0.20 mg cm−2of cathode catalyst loading. Test at 80 °C H2/air in MEA; fully humidified with total outlet pressure of 150 kPa; an anode stoichiometry of 2; and a cathode stoichiometry of 2 for air. The inset of each figure indicates the 3 difference between the power densities of MEAs with a conventional electrode and an IO electrode. Figure 5c,d (0.12 mg Pt cm −2 and 0.20 mg Pt cm −2 , respectively) were obtained from the US Department of Energy’s reference conditions with air. The polarization curves in the presence of oxygen, which show remarkably high power densities, are shown in Supplementary Fig. S6 . The performances of IO electrode-based MEAs in PEMFCs are higher than those of conventional MEAs with a similar Pt loading because of morphological advantages, enhanced effective diffusivity from the open electrode surface and interconnected pore architecture. All of these characteristics result in uncomplicated access of the reactant to the catalyst. The current density for the conventional MEA was 235 mA cm −2 ; this was measured for a catalyst loading of 0.12 mg cm −2 at 0.6 V under fully humidified operating conditions ( Fig. 5a ). The equivalent current measured under the same conditions for an IO electrode-based MEA with a similar Pt loading was 440 mA cm −2 (185% higher). In the case where the measurements were carried out under standard conditions with H 2 /air ( Fig. 5c,d ), the performances of the IO electrode-based MEAs were also better. The IO electrode fuel cell shows a slightly higher maximum power density and has a common configuration with a lower catalyst loading ( Fig. 5c ). In contrast, when a thicker electrode is used, the differences become more pronounced ( Fig. 5d ). This is because concentration losses due to mass transport of reactants and products increase in a thicker electrode. Specifically, a thicker electrode imposes a greater distance that reactants must diffuse through in order to reach the catalyst layer where the reactions occur. Likewise, a thicker electrode requires that products must diffuse over a greater distance to be removed from the fuel cell. The inset of each figure in Fig. 5 undoubtedly shows that the difference between the power densities of the two MEAs is significant for voltages under 0.7 V, but once the latter value is reached, the unit cells experience deficient oxygen transfer in the MEAs. On the contrary, by inspection of the open-circuit voltage to 0.7 V, the difference is not notable because those potentials are in the charge transfer-controlled region. Therefore, the PEMFC performances in the low-current region are nearly the same in both unit cells. However, the depletion of the reactant was reduced by their morphological advantages (for example, easy access to relatively large surface areas, highly open, low-tortuosity structures and interconnected macropores of the IO electrode), which resulted in a higher power density of the MEA containing the IO electrode in the high-current region. Figure 5: Polarization curves of IO electrode-based MEAs. ( a ) Using a fully humidified H 2 /O 2 supplement and maintained at 80 °C. ( b ) Under ambient humidity and room temperature condition. For both MEAs, the cathode catalyst loading was ~0.12 mg cm −2 . ( c ) Polarization curves from US Department of Energy’s reference conditions with 0.12 mg cm −2 and ( d ) 0.20 mg cm −2 of cathode catalyst loading. Test at 80 °C H 2 /air in MEA; fully humidified with total outlet pressure of 150 kPa; an anode stoichiometry of 2; and a cathode stoichiometry of 2 for air. The inset of each figure indicates the 3 difference between the power densities of MEAs with a conventional electrode and an IO electrode. Full size image The electrochemical surface area (ECSA) of the Pt catalyst was determined using hydrogen desorption areas from the cyclic voltammograms ( Supplementary Fig. S7 ), and then calculating the effects of factors such as Pt loading in the electrode, the amount of charge required for hydrogen desorption and the charge required to oxidize a monolayer of H (see Supplementary Note 1 for details) [53] . Our calculations determined that the ECSA of the IO electrode-based MEA was 24.13 m 2 g −1 . The geometric surface area (GSA) of the IO electrode-based MEA was estimated to be 40.04 m 2 g −1 , by taking into account the total number of 500 nm spheres in the IO electrode, both inside and outside areas of the sphere and the roughness factor of the sphere’s surface. The ECSA of the conventional MEA, on the other hand, was 57.01 m 2 g −1 . Furthermore, the particle sizes of the commercial Pt/C catalysts used in this work were in the range 2–4 nm and the GSA of the commercial Pt/C catalyst was 93 m 2 g −1 (see Supplementary Note 1 for details) [54] . The different ratios of the ECSA to GSA; that is, Pt utilization, for the catalysts are listed in Table 1 . In general, the GSA increases with decreasing grain particle size, thus the GSA and ECSA for a conventional MEA were higher than those for the IO electrode-based MEA. However, a higher ECSA does not always represent a better performance under actual fuel cell operating conditions. More importantly, the concept of GSA, ECSA and Pt utilization in this study only accounts for hydrogen adsorption/desorption reactions related to catalytic capacity, but excludes overall process parameters such as gas diffusion, ionic conduction path, proton conductivity, water and mass transfer in the MEAs; furthermore, any kinetic parameter was not included in the concept of Pt utilization as shown in Table 1 . This suggests that the IO electrode-based MEA could exhibit further improved performance even though its Pt utilization is nearly the same as that of conventional MEA. In addition, the active sites that participated in oxygen reduction at the Pt surface were well distributed over the electrode than those in the conventional MEA; the relationship between morphology and performance of the MEA is thus confirmed by these experimental data. Table 1 Structures and electrochemical properties of IO electrodes. Full size table Fuel cell losses are divided into three categories: activation, ohmic and concentration losses (or mass transfer losses). Although mass transfer loss occurs over the entire range of current density, it becomes prominent in the high limiting current region (lower potential region). Accordingly, polarization in the high-current density region represents mass transfer loss. The IO electrode-based MEA exhibited better performance than the conventional MEA, especially in the high-current region, at ambient humidity, owing to the enhanced mass transfer in the IO-MEA, and better water management, as explained below. In fuel cells, the effective porosity is more important than the total porosity. The effective porosity includes only the pore space that is interconnected and opens to the surface, such as that in an inverse opal structure. Theoretically, i=nFJ diff , where i is the fuel cell operating current and J diff is the diffusional flux. The J diff of the IO electrode is larger than that of the conventional MEA because of the IO electrode’s increased effective porosity and decreased diffusion layer thickness ( δ ). Therefore, it is possible to simultaneously achieve improved fuel cell operating current density ( i ) and limited current density ( i L ). In addition, enhanced mass transport may lead to superior water management. The effect of better water balance ability is clearly demonstrated under low-humidity conditions such as those shown in Fig. 5b , which are similar to conditions in a micro fuel cell. Hence, enhanced mass transfer and water management can be demonstrated by comparing the performances of the MEAs under conditions with and without further humidification. The water produced, which diffuses from cathode to anode, is driven by the water concentration gradient through the membrane (back diffusion). The water keeps the electrolyte sufficiently moist so that it retains its ionic conductivity. When water is deficient, better water management of the IO electrode more easily facilitates back diffusion and prevents a reduced cell performance. In particular, under ambient humidity at room temperature, the current density measured at 0.6 V for a conventional MEA (in the high-current density region) decreases rapidly from 666 to 367 mA cm −2 (45% loss), whereas that for the IO electrode-based MEA decreases from 790 to 495 mA cm −2 (37% loss, Fig. 5b ). These results demonstrate that the IO electrode-based MEA has a superior water transport capability that results from its highly open and low-tortuous structure and short diffusion pathway. Ordered meso-structured materials such as Pt or MoS 2 can improve both the activity and stability of the catalyst, but the enhancement of mass transfer has not yet been clearly demonstrated [55] , [56] . As reactants and products are mainly transferred through macro-sized secondary pores, and the mass transfer of MEA in a single cell is dominated by these secondary pores [57] . For that reason, IO electrodes with ordered macropore structures show better performance and more effective water management in practical fuel cell devices. Further, the open-circuit voltage of the IO electrode was 0.982 V, whereas that of the conventional MEA was 0.935 V under ambient humidity and room temperature conditions. This difference suggests that the mixed cathode potential for either the reactions between the Pt surface and O 2 , or from impurity oxidation [58] at the IO electrode, is lower than that for a conventional MEA. Thus, it is feasible to directly apply an inverse opal structure as an MEA electrode in PEMFCs. More importantly, the IO electrode has a much lower Pt loading and its performance is significantly better than that of general direct methanol fuel cells under similar operating conditions, for example, ambient humidity and heating. Thus, the IO electrode offers a promising MEA structure for use in micro fuel cell applications because the IO electrode fuel cell requires neither a complicated subsystem nor a balance of plant, unlike other fuel cell systems. We have demonstrated an approach for the facile and direct application of a large-area (5 cm 2 of active area) IO Pt electrode in a practical MEA device, without any additional transfer process required at the electrodes. An unsophisticated pretreatment process was required to adjust the substrate to enable PS bead deposition onto the rough substrate surface. Owing to their open and interconnected pore architecture, the IO electrodes maintained a good effective porosity, effective catalyst utilization and mass transfer, and satisfactory water management, while the concentration loss was minimized. Further, we have reported the unique performance of a single cell that features an inverse opal structure entirely within an MEA. Furthermore, the inverse-opal-structure Pt catalyst layer was free from carbon corrosion problems, as the electrode was neither based on carbon materials nor on carbon-based supports. It is expected that improved performance can be achieved by decreasing the Pt particle size and by optimizing the pore size. Moreover, with our approach, it is possible to vary both the colloidal size and species, and to use a non-precious metal alloy precursor. However, achieving high-performance PEMFCs with an IO electrode is not the only purpose of this study; discovering alternative, equally promising applications in electrochemical devices is another important purpose. Materials and characterization Commercially available solvents and reagents were used without further purification unless otherwise noted. Carboxylated PS latex particles with a mean diameter of 520 nm in a 10 wt% aqueous suspension were obtained from Thermo Fisher Scientific, Inc. The surface morphology and thickness of the PS colloidal crystal template and the IO Pt electrode were characterized using FE-SEM (Carl Zeiss, SUPRA 55VP). Atomic force microscopy was carried out to identify the surface structure and roughness of the electrodes. XPS were obtained from an Al Kα source (ESCALAB 250 XPS spectrometer, VG Scientifics). Binding energies were calibrated with respect to C (1 s) at 285 eV. Experimental data were curve-fitted using AVANTAGE4.19 software. The Pt in the IO electrodes was examined using X-ray diffraction (Rigaku D-MAX2500 152-PC) with CuKα radiation (40 kV, 200 mA) at room temperature. The loading mass of Pt on the GDLs was estimated using ICP-optical emission spectroscopy, Varian 820-MS (Varian). Before analysis, the catalysts were dissolved in aqua regia for 24 h and then diluted to a certain concentration. Assembled single cells (CNL-PEM005-01, CNL Energy) were tested using the current-sweep-hold method with a fuel cell test system (CNL Energy). Cyclic voltammetry (CV) with a potentiostat/galvanostat (IM-6, Zahner) was used to determine the ECSA. Electrochemical measurements were carried out using an Autolab potentiostat (PGSTAT128N) in a standard three-compartment electrochemical cell with an IO electrode, Pt plate and saturated calomel electrode as the working, counter and reference electrodes, respectively. All potentials are quoted with respect to that of a normal hydrogen electrode, and all measurements were conducted at room temperature. Preparation of opal-structure PS template The substrate (GDLs) were soaked in a 1,2-ethanedithiol solution in ethanol (10 mM) for at least 12 h before PS bead deposition to enhance adhesion between the substrate and colloid; 0.36 g of the 0.5 wt% non-ionic surfactant (IGEPAL Co-30) and 80 ml of Milli-Q water were mixed together, and 0.5 g of PS suspension were added. The mixtures were then ultrasonicated for 30 min, placed in an oven,and dried at 65 °C for more than 2 days under a constant relative humidity. Fabrication of inverse-opal-structure Pt electrode Galvanostatic-pulsed electrodeposition of Pt onto the template was performed in a three-electrode cell with a Pt plate counter electrode and an Ag/AgCl reference electrode using an Autolab potentiostat (PGSTAT128N). The substrate, GDL (SGL 35BC carbon paper), was purchased from the SGL Group. The GDL substrate under the template served as the working electrode. Electrodeposition was carried out in a plating bath containing a solution of 10 mM H 2 PtCl 4 dissolved in 10 mM KCl. The duty cycle (%) of the pulsed electrodeposition is defined as ( θ 1 /( θ 1 + θ 2 )) × 100, where θ 1 =on-time and θ 2 =off-time. The morphology of the IO electrode changed with variations in the duty cycle and current density. The parameters chosen in this work were a peak current density of 50 mA cm −2 , an on-/off-time of 50/100 ms and a total charge of 4 C cm −2 . The actual amount of Pt deposited onto the GDL was ~0.12 mg cm −2 , as confirmed using ICP mass spectrometry. After deposition, PS particles were removed by soaking in toluene for 12 h. The GDL was removed from the solution and was washed with water. The electrode was heated in a furnace at 130 °C in air for 4 h to remove the water and the contaminants contained in the interstitial spaces of the inverse opal. During the second step, the electrode was heat-treated at 180 °C for 2 h under H 2 to remove any remaining organic solvent and to minimize Pt oxidation. The second step is optional. MEA fabrication The typical MEA fabrication procedure has been described elsewhere [6] , [7] . A Nafion 212 membrane (DuPont) was used for the ion-conducting membrane, which was immersed in a 2.5% H 2 O 2 solution at 80 °C for 1 h, and then rinsed in boiling deionized water for 1 h for purification. The membrane was then boiled in a 0.5 M H 2 SO 4 solution for 1 h and rinsed in deionized water for protonation. An IO electrode was used as the cathode and 40 wt% Pt/C (Johnson Matthey Co.) was used as the anode catalyst. The Pt/C catalyst was dispersed in a mixture of isopropyl alcohol, deionized water and perfluorosulfonic acid ionomer (Aldrich, 5 wt% Nafion ionomer) to prepare the catalyst ink. The latter was ultrasonicated for 15 min and sprayed onto the anode side of a Nafion 212 membrane. The volume of catalyst ink was controlled to deposit 0.12–0.20 mgPt·cm −2 in order to prepare the catalyst-coated membranes (CCMs). SGL 35BC carbon paper was used as a GDL, and it was placed on the anode side of the CCMs. The MEAs were inserted into a single-cell unit that had a graphite plate with a serpentine gas flow channel (5 cm 2 area). A single-cell unit was assembled with eight screws and a tightening torque of 8 N m ( Fig. 4 ). Activation and polarization tests of the assembled single cells were performed using the current-sweep-hold method with a fuel cell test system. The current was maintained for 10 min when the current density reached each of the following values, 0.5, 1.0, 1.5, 2.0, 2.5, 3 and 4 A cm −2 , during a 10 mA cm −2 s −1 current-sweep rate. During activation, the current was reset to 0 when the cell voltage reached 0.35 V. Polarization curves ( Fig. 5 ) were measured using the current-sweep method and the PEMFC test system. The test was conducted using fully humidified H 2 /O 2 (or air), which was supplied to the anode and cathode, respectively, during activation and the polarization tests. The total outlet pressure was 150 kPa with an anode stoichiometry of 2, a cathode stoichiometry of 9.5 for O 2 and an air stoichiometry of 2. The cell temperature was maintained at 80 °C during activation and at room temperature during the polarization test. The catalyst loading was 0.12 mg cm −2 . For the cathodic dead-end mode, the flow rate of O 2 was minimized and the outlet of the cell was closed. Electrochemical characterization The ECSA of the cathode catalyst layer was estimated using CV ( Supplementary Fig. S7 ). After the polarization test, the single cell was purged with humidified N 2 gas on both cell sides for 12 h to remove reactant gases. Humidified H 2 and N 2 gases (99.999%) were supplied to the anode and cathode sides, respectively, and the cell temperature was maintained at 30 °C to measure the CV after N 2 purging. The voltage sweep range of the CV was 0.05–1.20 V, and the scan rate was 100 mV s −2 . How to cite this article: Kim, O.-H. et al. Ordered macroporous platinum electrode and enhanced mass transfer in fuel cells using inverse opal structure. Nat. Commun. 4:2473 doi: 10.1038/ncomms3473 (2013).